Pyrimidine pool imbalance induced by BLM helicase deficiency contributes to genetic instability in Bloom syndrome Defects in DNA replication are associated with genetic instability and cancer development, as illustrated in Bloom syndrome. Features of this syndrome include a slowdown in replication speed, defective fork reactivation and high rates of sister chromatid exchange, with a general predisposition to cancer. Bloom syndrome is caused by mutations in the BLM gene encoding a RecQ helicase. Here we report that BLM deficiency is associated with a strong cytidine deaminase defect, leading to pyrimidine pool disequilibrium. In BLM-deficient cells, pyrimidine pool normalization leads to reduction of sister chromatid exchange frequency and is sufficient for full restoration of replication fork velocity but not the fork restart defect, thus identifying the part of the Bloom syndrome phenotype because of pyrimidine pool imbalance. This study provides new insights into the molecular basis of control of replication speed and the genetic instability associated with Bloom syndrome. Nucleotide pool disequilibrium could be a general phenomenon in a large spectrum of precancerous and cancer cells. Bloom syndrome (BS) is a rare autosomal recessive disorder characterized by marked genetic instability associated with predisposition to a wide range of cancers commonly affecting the general population [1] . BS is caused by mutations in the BLM gene, which encodes BLM, a RecQ 3′–5′ DNA helicase, indicating an essential role for BLM in maintaining genetic stability and preventing cancer [2] . In vitro , BLM unwinds DNA structures mimicking replication forks and homologous recombination intermediates [3] . The specific functions of BLM remain unclear, but it is widely thought that BLM is involved in restarting blocked replication forks [4] , [5] . In the absence of BLM, cells display a high rate of sister chromatid exchanges (SCEs), pathognomonic for BS [6] . BS cells also display a slowing of replication fork progression associated with endogenous activation of the ATM-Chk2-γH2AX pathway [4] , [5] . This pathway is activated in precancerous lesions and is thought to be a part of an antitumorigenesis barrier [7] , [8] . This barrier is based on DNA replication stress, leading to activation of the DNA damage checkpoint and, thus, apoptosis or cell cycle arrest [7] , [8] . BS cells may therefore be in a precancerous state. Our working hypothesis is that BLM deficiency results in a global 'SOS-like' cellular response, facilitating progression through the antitumorigenesis barrier potentially involved in carcinogenesis in the general population [9] . Thus, identification of the genes and pathways deregulated in the absence of BLM may facilitate the establishment of a molecular signature of the precancerous state. Deoxyribonucleoside triphosphate (dNTP) levels are also of major importance for maintaining genomic integrity. Indeed, nucleotide pool imbalance, particularly for the pyrimidine pools, is known to result in genetic instability and oncogenic transformation [10] , [11] . Pyrimidine biosynthesis occurs through the de novo pathway, in which nucleotides are synthesized from small metabolites, or the salvage pathway, which recycles nucleosides and nucleotides [12] . In mammalian cells, deficiencies of many of the enzymes involved in the two pyrimidine biosynthesis pathways, such as thymidine kinase, dTMP synthase, dCTP kinase, CTP synthase and dCMP deaminase, have been associated with the induction of mutations, DNA breaks, sensitization to DNA-damaging agents, increase in the rate of homologous recombination and chromosomal abnormalities [10] , [11] . We report here that BLM deficiency leads to cytidine deaminase (CDA) downregulation, resulting in pyrimidine pool disequilibrium, accounting for the slowing of replication fork progression and contributing to the increase in SCE frequency associated with the BS phenotype. BLM deficiency is associated with a strong CDA defect For the identification of genes specifically deregulated in the absence of BLM, we performed a microarray analysis comparing the transcriptome of wild-type HeLa cells with that of HeLa cells in which BLM was downregulated [13] , and the transcriptome of the GM8505B BS cell line (BS) with that of its BLM-complemented counterpart (green fluorescent protein (GFP)-BLM). We identified 77 candidate genes for which regulation was potentially modified in the same way in both HeLa cells depleted of BLM and in BS cells ( Supplementary Table S1 ). One of these genes, encoding CDA (EC 3.5.4.5; locus 1p36.2-p35), particularly attracted our attention. CDA is an enzyme of the pyrimidine salvage pathway catalysing the hydrolytic deamination of cytidine (C) and deoxycytidine (dC) to uridine (U) and deoxyuridine (dU), respectively [14] . We confirmed that CDA mRNA and protein levels were strongly reduced in BS cells and in BLM-downregulated HeLa cells, and in HEK 293 human embryonic kidney cells depleted of BLM ( Fig. 1a ). The expression of a functional BLM protein (GFP-BLM) in BS cells was sufficient to restore CDA expression ( Fig. 1a ). By contrast, expression of a BLM protein with an inactive helicase domain but a functional DNA-binding domain (GFP-BLMI841T) [15] in BS cells failed to rescue CDA gene expression ( Fig. 1a ), demonstrating the requirement of BLM helicase activity for CDA gene expression. We inserted the human CDA promoter into a luciferase vector and showed that the CDA promoter was significantly less active in the absence of BLM or of its helicase activity ( Fig. 1b ), demonstrating the requirement of BLM helicase activity for correct CDA expression and, thus, the direct or indirect involvement of this activity in regulation of the CDA promoter. 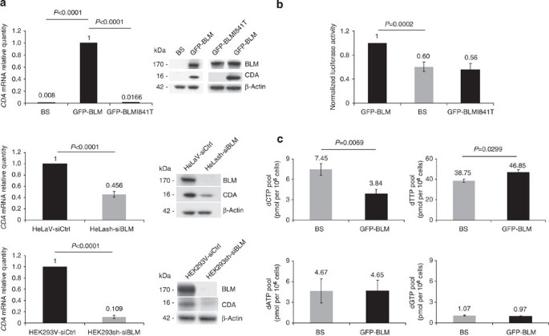Figure 1: BLM deficiency is associated with CDA deficiency and pyrimidine pool imbalance. (a) CDA mRNA and protein levels determined by real-time quantitative PCR and western blotting, respectively, in BS, GFP-BLM and GFP-BLMI841T cells (upper panels), in HeLash-siBLM and HeLaV-siCtrl cells (middle panels) and in human embryonic kidney HEK293sh-siBLM and HEK293V-siCtrl cells (lower panels). Error bars represent the s.e.m. of three independent experiments. The significance of differences was assessed by Student'st-tests. (b) Analysis ofCDApromoter activity based on the luciferase assay in BS, GFP-BLM and GFP-BLMI841T cells. Firefly luciferase activity was normalized with respect to that of theRenillaluciferase expressed from a control vector introduced by co-transfection. Error bars represent the s.e.m. of seven independent experiments. The significance of differences was assessed by Student'st-tests. (c) Deoxycytidine triphosphate (dCTP) and deoxythymidine (dTTP) levels in BS and GFP-BLM cells. Error bars represent the s.e.m. of seven independent experiments. The significance of differences was assessed by Student'st-tests (upper panels). Deoxyadenosine triphosphate (dATP) and deoxyguanosine triphosphate (dGTP) levels in BS-GFP and GFP-BLM cells. Error bars represent the s.e.m. of three independent experiments (lower panels). Figure 1: BLM deficiency is associated with CDA deficiency and pyrimidine pool imbalance. ( a ) CDA mRNA and protein levels determined by real-time quantitative PCR and western blotting, respectively, in BS, GFP-BLM and GFP-BLMI841T cells (upper panels), in HeLash-siBLM and HeLaV-siCtrl cells (middle panels) and in human embryonic kidney HEK293sh-siBLM and HEK293V-siCtrl cells (lower panels). Error bars represent the s.e.m. of three independent experiments. The significance of differences was assessed by Student's t -tests. ( b ) Analysis of CDA promoter activity based on the luciferase assay in BS, GFP-BLM and GFP-BLMI841T cells. Firefly luciferase activity was normalized with respect to that of the Renilla luciferase expressed from a control vector introduced by co-transfection. Error bars represent the s.e.m. of seven independent experiments. The significance of differences was assessed by Student's t -tests. ( c ) Deoxycytidine triphosphate (dCTP) and deoxythymidine (dTTP) levels in BS and GFP-BLM cells. Error bars represent the s.e.m. of seven independent experiments. The significance of differences was assessed by Student's t -tests (upper panels). Deoxyadenosine triphosphate (dATP) and deoxyguanosine triphosphate (dGTP) levels in BS-GFP and GFP-BLM cells. Error bars represent the s.e.m. of three independent experiments (lower panels). Full size image CDA has an essential role in maintaining the cellular pool of nucleotides, which is crucial for genome stability. Indeed, an imbalance in the nucleotide pools is highly mutagenic in mammalian cells [16] , and BS cells display a mutator and hyper-Rec phenotype [6] , [17] . The purine pools were not affected in BS cells, whereas the pyrimidine pools were significantly unbalanced ( Fig. 1c ). Indeed, BS cells had about twice as much dCTP and a slightly lower level of dTTP than GFP-BLM cells ( Fig. 1c ). Moreover, expression of the GFP-BLMI841T non-functional protein in BS cells, which was not able to rescue CDA gene expression ( Fig 1a ), also failed to normalize the dCTP pool size ( Supplementary Fig. S1 ). CDA expression partially rescues cellular BS phenotype Stable expression of the CDA gene in BS cells (BS-CDA) was sufficient to restore a dCTP pool similar to that of GFP-BLM cells ( Fig. 2a ), demonstrating the direct responsibility of the CDA defect for the pyrimidine pool imbalance observed in BLM-deficient cells. CDA expression in BS cells also decreased the frequency of SCE by 25% ( P =0.0015, Student's t -test), reflected in a great decrease in the number of cells with high levels of SCE ( Fig. 2b ), suggesting a direct relationship between the high rate of SCE observed in BS cells and nucleotide pool disequilibrium. Addition of 500 μM dC to the culture medium of GFP-BLM cells led to a 1.75 times increase in dCTP pool size ( Fig. 2c ) and ∼ 42% increase in SCE frequency ( P =0.0327, Student's t -test; Fig. 2d ), confirming that nucleotide pool disequilibrium promotes an increase in SCE frequency. CDA expression in BS cells also increased colony-forming efficiency significantly ( Fig. 2e ). Moreover, CDA expression in BS cells was sufficient to increase replication fork speed, by up to 24%, restoring fork velocity to levels similar to those in GFP-BLM cells ( Fig. 2f ). These results suggest that the slowdown of replication speed in BS cells could be the consequence of the pyrimidine pool imbalance. 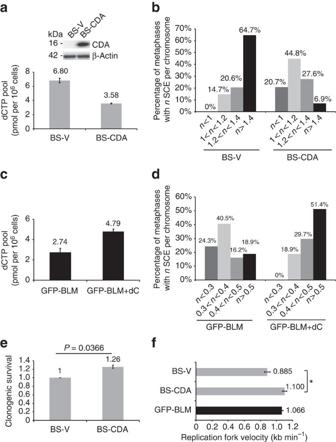Figure 2: CDA expression in BLM-deficient cells partially complements BS phenotype. (a) dCTP pool level in BS-V and BS-CDA cells and CDA expression assessed by immunoblotting. Error bars represent the range of two independent experiments. (b) Percentage of metaphases withnSCE per chromosome from BS-V and BS-CDA cells. In all, 40–50 metaphases from three independent experiments were analysed for each condition. (c) dCTP pool level in GFP-BLM cells untreated or treated with dC. Error bars represent the range of two independent experiments. (d) Percentage of metaphases withnSCE per chromosome from GFP-BLM cells untreated or treated with dC. In all, 40–50 metaphases from three independent experiments were analysed for each condition. (e) BS-V or BS-CDA cells were plated in triplicate at three dilutions (200, 400 and 600 cells). Error bars represent the s.e.m. of three independent experiments. The significance of differences was assessed by Student'st-tests. (f) Replication fork velocity in BS-V, BS-CDA and GFP-BLM cells. Error bars represent the range of two independent experiments. Mann–Whitney statistical tests have been performed on the total number of fork analysed from the two experiments (BS-V,n=880; BS-CDA,n=568; and GFP-BLM:n=800). Asterisk indicates aP-value <0.00001. Figure 2: CDA expression in BLM-deficient cells partially complements BS phenotype. ( a ) dCTP pool level in BS-V and BS-CDA cells and CDA expression assessed by immunoblotting. Error bars represent the range of two independent experiments. ( b ) Percentage of metaphases with n SCE per chromosome from BS-V and BS-CDA cells. In all, 40–50 metaphases from three independent experiments were analysed for each condition. ( c ) dCTP pool level in GFP-BLM cells untreated or treated with dC. Error bars represent the range of two independent experiments. ( d ) Percentage of metaphases with n SCE per chromosome from GFP-BLM cells untreated or treated with dC. In all, 40–50 metaphases from three independent experiments were analysed for each condition. ( e ) BS-V or BS-CDA cells were plated in triplicate at three dilutions (200, 400 and 600 cells). Error bars represent the s.e.m. of three independent experiments. The significance of differences was assessed by Student's t -tests. ( f ) Replication fork velocity in BS-V, BS-CDA and GFP-BLM cells. Error bars represent the range of two independent experiments. Mann–Whitney statistical tests have been performed on the total number of fork analysed from the two experiments (BS-V, n =880; BS-CDA, n =568; and GFP-BLM: n =800). Asterisk indicates a P -value <0.00001. Full size image CDA downregulation reproduces part of the BS phenotype The short interfering RNA (siRNA)-mediated downregulation of CDA in GFP-BLM cells increased the frequency of SCE by 46% ( P =0.0134, Student's t -test), reflecting a significant increase in the number of cells with a high SCE frequency ( Fig. 3a ). By contrast, transient transfection of BS cells (with no detectable CDA expression) with siRNAs specific for CDA had no effect on SCE level ( Supplementary Fig. S2 ). CDA downregulation in HeLa cells and in BLM-downregulated HeLa cells (in which CDA downregulation was not complete as seen in Fig. 1a ) also significantly increased the number of cells with a high SCE frequency ( Fig. 3b ). Moreover, CDA downregulation significantly decreased replication fork velocity in GFP-BLM cells, but not in BS cells ( Fig. 3c ). Thus, the level of CDA gene expression influences both SCE frequency and the speed of the replication fork, CDA downregulation being associated with an increase in the level of SCE and a decrease in the replication fork velocity. 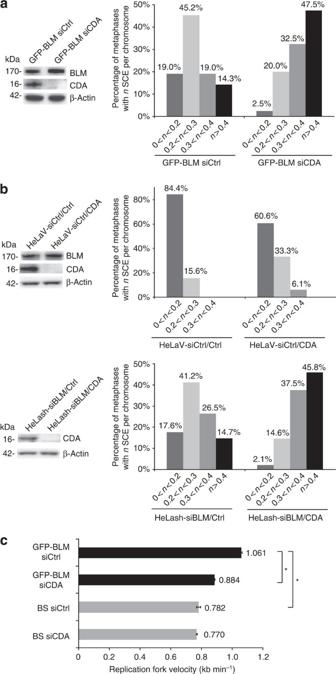Figure 3: siRNA-mediated CDA depletion partially reproduces BS phenotype. (a) Percentage of metaphases withnSCE per chromosome from GFP-BLM cells transfected with the indicated siRNAs. In all, 40–50 metaphases from three independent experiments were analysed for each condition. CDA levels were assessed by immunoblotting. (b) Percentage of metaphases withnSCEs per chromosome from HeLaV-siCtrl and HeLash-siBLM cells transiently transfected with the indicated siRNAs. CDA protein levels were assessed by immunoblotting. About 40–50 metaphases from two independent experiments were analysed for each condition. (c) Replication fork velocity in GFP-BLM and BS cells transfected with the indicated siRNAs. Error bars represent the range of two independent experiments. Mann–Whitney statistical tests have been performed on the total number of forks analysed from the two experiments (GFP-BLM siCtrl,n=312; GFP-BLM siCDA,n=452; BS siCtrl:n=459; and BS siCDA,n=467). Asterisks indicate aP-value <0.00001. Figure 3: siRNA-mediated CDA depletion partially reproduces BS phenotype. ( a ) Percentage of metaphases with n SCE per chromosome from GFP-BLM cells transfected with the indicated siRNAs. In all, 40–50 metaphases from three independent experiments were analysed for each condition. CDA levels were assessed by immunoblotting. ( b ) Percentage of metaphases with n SCEs per chromosome from HeLaV-siCtrl and HeLash-siBLM cells transiently transfected with the indicated siRNAs. CDA protein levels were assessed by immunoblotting. About 40–50 metaphases from two independent experiments were analysed for each condition. ( c ) Replication fork velocity in GFP-BLM and BS cells transfected with the indicated siRNAs. Error bars represent the range of two independent experiments. Mann–Whitney statistical tests have been performed on the total number of forks analysed from the two experiments (GFP-BLM siCtrl, n =312; GFP-BLM siCDA, n =452; BS siCtrl: n =459; and BS siCDA, n =467). Asterisks indicate a P -value <0.00001. Full size image Addition of dU partially rescues BS phenotype Finally, we found that the addition of 25 μM dU (the final CDA product) or thymidine (T) to the culture medium led to ∼ 40% decrease in SCE frequency in BS cells ( Fig. 4a ). As the addition of dU at this concentration had no effect on residual SCE frequency in GFP-BLM cells or on the quality of the differential labeling of sister chromatids in either cell line, and did not modify the rate of 5-bromodeoxyuridine incorporation into DNA ( Supplementary Fig. S3 ), we concluded that the addition of dU or T mimicked the activity of CDA, thus accounting for the observed decrease in SCE frequency in BS cells ( Fig. 4a ). Moreover, dU addition led to an 18.2% increase in fork velocity in BS cells but had no effect on fork velocity in GFP-BLM cells ( Fig. 4b ). The number of asymmetric replication bubbles in BS cells, reflecting the number of arrested forks [5] , was not affected by dU addition ( Fig. 4c ). These results show that the addition of dU efficiently decreased the frequency of SCE and restored fork velocity in BS cells (although not to the same extent as CDA expression), demonstrating that the contribution of the CDA defect to the BS phenotype results from pyrimidine pool disequilibrium. These results also make it possible to distinguish between the replication fork velocity and fork restart as two independent events, both affected by BLM helicase deficiency, through nucleotide pool disequilibrium in the case of the replication fork velocity. 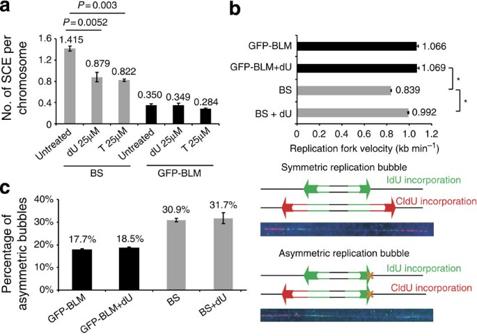Figure 4: The BS phenotype is partially complemented by dU or T. (a) SCE frequencies in BS and GFP-BLM cell lines untreated or treated with dU or T (about 1,800 chromosomes analysed for each condition). Error bars represent the s.e.m. of three independent experiments. The significance of differences was assessed by Student'st-tests. (b) Replication fork velocity in GFP-BLM and BS cell lines untreated or treated with dU. Error bars represent the range of three independent experiments. Mann–Whitney statistical tests have been performed on the total number of forks analysed from the three experiments (GFP-BLM,n=530; GFP-BLM+dU,n=642; BS,n=858; and BS+dU,n=440). Asterisks indicate aP-value <0.00001. (c) Percentage of asymmetric replication bubbles in BS and GFP-BLM cell lines untreated or treated with dU, and examples of symmetric and asymmetric bubbles (70–130 replication bubbles analysed for each condition). CldU, chlorodeoxyuridine; IdU, iododeoxyuridine. Error bars represent the range of two independent experiments. Figure 4: The BS phenotype is partially complemented by dU or T. ( a ) SCE frequencies in BS and GFP-BLM cell lines untreated or treated with dU or T (about 1,800 chromosomes analysed for each condition). Error bars represent the s.e.m. of three independent experiments. The significance of differences was assessed by Student's t -tests. ( b ) Replication fork velocity in GFP-BLM and BS cell lines untreated or treated with dU. Error bars represent the range of three independent experiments. Mann–Whitney statistical tests have been performed on the total number of forks analysed from the three experiments (GFP-BLM, n =530; GFP-BLM+dU, n =642; BS, n =858; and BS+dU, n =440). Asterisks indicate a P -value <0.00001. ( c ) Percentage of asymmetric replication bubbles in BS and GFP-BLM cell lines untreated or treated with dU, and examples of symmetric and asymmetric bubbles (70–130 replication bubbles analysed for each condition). CldU, chlorodeoxyuridine; IdU, iododeoxyuridine. Error bars represent the range of two independent experiments. Full size image This study demonstrates for the first time that BLM deficiency leads to CDA downregulation, resulting in pyrimidine pool disequilibrium and accounting, in part, for the BS phenotype. However, it remains unclear how BLM controls CDA expression. We demonstrate here that the helicase activity of BLM regulates CDA promoter function either directly or indirectly. The preferred substrates for the recombinant BLM protein are G-quadruplex structures [18] , [19] . However, we identified no potential intramolecular G-quadruplex-forming sequences or particular sequences likely to form secondary structures in the CDA promoter (using Quad Parser, website http://www.quadruplex.com ), suggesting that CDA expression is not repressed by secondary structures formed in the absence of BLM. Furthermore, in our microarray study, none of the genes with deregulated expression in the absence of BLM encoded a known transcriptional factor ( Supplementary Table S1 ). Another possibility is that BLM directly targets certain promoters, as reported for the WRN helicase [20] . The key findings of this work are that the defect in replication fork speed and, a fraction of the increase in SCE frequency in BS cells are the consequences of a cascade reaction in which the defect in BLM helicase activity leads to a CDA expression defect that in turn provokes a pyrimidine pool disequilibrium. Importantly, replication fork progression defect can be rescued and the rate of SCEs reduced by 25–40% by acting on the nucleotide pool, without restoring BLM activity. Indeed, addition of dU, the final CDA product, was found to be sufficient to restore the replication fork velocity and to decrease significantly the level of SCEs in BLM-deficient cells. These data highlight the direct mechanistic connection between the replication defect, part of the increase in SCE and pyrimidine pool disequilibrium in BS cells. Decrease in the fork velocity because of the nucleotide pool disequilibrium may lead to replication stress and, thus, to an increase in replication-associated DNA breaks, accounting in part for SCE formation. These data indicate that the high frequency of SCEs in BS cells has at least two different origins: 60–75% of SCEs may reflect the restarting of blocked replication forks through RAD51-mediated homologous recombination [13] , as proposed in several models [9] , [21] , [22] . The remaining 25–40% of SCEs may reflect the repair of DNA breaks because of pyrimidine pool disequilibrium. This second type of SCEs may also be dependent on RAD51-dependent homologous recombination [13] . This study also demonstrates that CDA downregulation in BLM-expressing cells leads to a significant increase in SCE frequency and replication stress, potentially conferring a predisposition to cancer. A previous French study reported that 7% of adult patients with cancer treated with gemcitabine (5′-azacytidine, 2′,2′-difluorodeoxycytidine), a CDA substrate, had very low levels of CDA activity, rendering gemcitabine highly toxic [23] . We therefore suggest that CDA deficiency may be a marker of predisposition to cancer in the general population. Cell culture and treatments Cell lines were cultured in DMEM supplemented with 10% FCS. BS and GFP-BLM cells were obtained by transfecting BS GM08505B cells with the EGFP-C1 vector alone (Clontech) or with the same vector containing the full-length BLM cDNA [24] , respectively, using JetPEI reagent (Ozyme). After 48 h, selection with 800–1,600 μg ml −1 G418 (PAA) was applied. Individual colonies were isolated and cultured in medium containing 500 μg ml −1 G418. GFP-BLMI841T cells were obtained by transfecting BS GM08505B cells as described above, with the EGFP-C1 vector containing the full-length BLM cDNA mutated at codon 841. HeLaV and HeLashBLM cells, HEK293V and HEK293shBLM cells were obtained by transfecting cells with an empty pSM2 vector or with the same vector encoding a short hairpin RNA sequence directed against BLM (Open Biosystems, clone V2HS-89234), respectively, using JetPEI reagent. After 48 h, selection with 1–5 μg ml −1 puromycin (Invivogen) was done. Individual colonies were isolated and cultured in medium containing 0.5 μg ml −1 puromycin. BS-V and BS-CDA cell lines were obtained by transfecting BS cells with an empty pCI-puro vector [25] , or with the same vector containing the full-length CDA cDNA (NM001785), using JetPEI reagent. After 48 h, selection was carried out with 0.2 μg ml −1 puromycin (Invivogen) and 500 μg ml −1 G418 (Invitrogen). Individual colonies were isolated and maintained in culture with 0.1 μg ml −1 puromycin and 500 μg ml −1 G418. For siRNA transfection assays, 3×10 5 to 4×10 5 HeLa or HEK cells or 8×10 5 to 9×10 5 BS or GFP-BLM cells were used to seed the wells of a six-well plate. Cells were transfected with an siRNA specific for BLM or CDA (ON-TARGETplus SMARTpool, Dharmacon) or negative control siRNAs (ON-TARGETplus siCONTROL Non Targeting Pool, Dharmacon; 100 nM final concentration) for 48 h for BLM, or twice successively, for a total of 120 h for CDA using DharmaFect (Dharmacon). Deoxyribonucleosides (Sigma) were added to the cell culture medium at a final concentration of 500 μM (dC) and 25 μM (dU, T) for 96 h (2×48 h). Transcriptomic analysis with Affymetrix microarrays Analysis was performed on BS, GFP-BLM, HeLaV-siCtrl and HeLash-siBLM cell lines. For each cell line, three independent total RNA samples were extracted using the RNeasy system (Qiagen). Fragmented biotinylated antisense RNA was generated and hybridized to Affymetrix Human Genome U133 Plus 2.0 Arrays. After hybridization, arrays were scanned following guidelines from Affymetrix ( http://www.affymetrix.com ). These arrays contain ∼ 54,000 probesets, representing ∼ 47,000 transcripts. Statistical analysis of microarray expression experiments was performed as previously described [26] using a P -value cutoff of 0.05. Raw and normalized transcriptomic data are available at the Institut Curie microarray dataset repository ( http://microarrays.curie.fr/ . Direct link: http://microarrays.curie.fr/publications/UMR3348/pyrimidine-bloom-syndrome/ ). Plasmid construction and site-directed mutagenesis Site-directed mutagenesis was carried out in the EGFP-C1 vector containing the full-length BLM cDNA: Ile-841 was mutated with the QuikChange XL site-directed mutagenesis kit (Stratagene) according to the manufacturer's instructions. Primer 1 (5′-CCCAGGGTACAGAAGGACACCCTGACTCAGCTGAAG-3′) and primer 2 (5′-CTTCAGCTGAGTCAGGGTGTCCTTCTGTACCCTGGG-3′) were used. Reverse transcription and real-time quantitative PCR Total RNA was extracted with RNeasy Mini kit (Qiagen) including a DNAse digestion step. RNA quality was assessed with the Experion system (BioRad), and cDNAs were synthesized with 250 ng of random hexamers (Invitrogen), 2 μg of RNA and Superscript II reverse transcriptase (Invitrogen). Quantitative PCR experiments were performed according to the MIQE Guideline [27] . Amplification mixtures contained the cDNA template (1/100 dilution), SYBR Green Supermix 1× (BioRad) and 300 nM forward and reverse primers. Amplification was performed with the CFX96 detection system (BioRad). The relative quantities of the CDA and BLM cDNAs were normalized against four reference genes ( RPL32 , HPRT1 , HMBS and SDHA ) chosen on the basis of their low M -value [28] . The primer sequences for BLM, RPL32, HPRT1, HMBS and SDHA have been described in previous publications [28] , [29] , [30] . CDA primer sequences: primer 1 (5′-CCCTACAGTCACTTTCCTG-3′) and primer 2 (5′-CGGGTAGCAGGCATTTTCTA-3′). Western blot analysis and antibodies Cells were lysed in 350 mM NaCl, 50 mM Tris–HCl, pH7.5, 1% NP-40 and protease inhibitors (Roche), sonicated and heated at 70 °C for 10 min. Samples equivalent to 25 μg of protein were subjected to electrophoresis in NuPAGE Novex 4–12% Bis-Tris pre-cast gels (Invitrogen). The procedures used for gel electrophoresis and immunoblotting have been described elsewhere [13] . Primary and secondary antibodies were used at the following concentrations: rabbit anti-BLM antibody (1:1,000; ab476 from Abcam); rabbit anti-CDA antibody (1:500; ab56053 from Abcam); rabbit anti-β-actin antibody (1:10,000; Sigma); and horseradish peroxidase-conjugated goat anti-rabbit IgG (1:5,000; Santa Cruz Biotechnology). dNTP assays Assays were performed as previously described [31] . Briefly, dNTPs were extracted from fresh cell pellets (10–40×10 6 cells) in 0.6 M trichloroacetic acid and 15 mM MgCl 2 . Extracts were neutralized and used immediately or stored at −80 °C. For each dNTP assay, an oligonucleotide template primer was designed [31] , and DNA polymerization reactions were carried out with Sequenase (USB Corporation) and a radiolabeled nucleotide (Perkin Elmer) on samples or on dNTP standard solutions (0–4 pM). Samples were spotted on to DE81 membranes (Whatman), which were washed with 5% (w/v) Na 2 HPO 4 (Sigma) and counted in a liquid scintillation counter. dTTP and dCTP pools were determined in GFP-BLM cells treated with 2 mM hydroxyurea (Sigma) for 2 h as a positive control for the dNTP assay ( Supplementary Fig. S4 ). SCE assays Cells were transferred to slides and cultured in the presence of 10 μM 5-bromodeoxyuridine (BrdU) (Sigma) during two cell divisions. After 40–48 h, colchicine (Sigma) was added (0.1 μg ml −1 ) and the cells were incubated for 1 h. Cells were then incubated in hypotonic solution (1:5 (vol/vol) FCS-distilled water) and fixed with a 3:1 (vol/vol) mixture of methanol-acetic acid. Cells were then stained by incubation with 10 μg ml −1 Hoechst 33258 (Sigma) in distilled water for 20 min, rinsed with 2×SSC (Euromedex), exposed to ultraviolet light at 365 nm at a distance of 10 cm for 105 min, rinsed in water, stained by incubation with 2% Giemsa solution (VWR) for 16 min, rinsed in water, dried and mounted. Chromosomes were observed with a Leica DMRB microscope at ×100 magnification. Metaphases were captured with a SONY DXC 930 P camera and SCEs were analysed. DNA molecular combing Asynchronous populations of cells were labeled by incubation for 40 min with 100 μM IdU (Sigma-Aldrich), washed with medium at 37 °C and then labeled by incubation for 40 min with 100 μM CldU (Sigma-Aldrich). The DNA solution was prepared as previously described [5] , and DNA was combed on silane-treated coverslips with a combing apparatus (Genomic Vision). Coverslips with combed DNA were baked overnight at 60 °C and incubated in 0.5 M NaOH–1 M NaCl solution for 15 min, with gentle shaking, for DNA denaturation. Coverslips were washed several times in PBS and dried by successive incubations, for 5 min each, in 70, 90 and 100% ethanol. They were then incubated with the primary antibodies. All antibodies were diluted in BlockAid (Invitrogen). Coverslips were incubated at room temperature, first with 1/5 mouse anti-BrdU (BD Biosciences)+1/25 rat anti-CldU (ABserotec) for 1 h, then with 1/25 goat anti-mouse 488+1/25 Alexa Fluor goat anti-rat 555 antibodies (Invitrogen) for 40 min, followed by 1/50 mouse anti-ssDNA antibody (Millipore) for 40 min, then 1/25 rabbit anti-mouse 350 antibody (Invitrogen) for 30 min and finally with 1/25 goat anti-rabbit 350 antibody (Alexa Fluor, Invitrogen) for 30 min. Between incubations, coverslips were washed three times, for 5 min each, in PBS. Coverslips were mounted in Prolong Gold antifade reagent (Invitrogen). Images were acquired with a Leica DM RXA microscope equipped with a motorized XY stage, using a ×40 PlanApo N.A. 1.25 objective and a CoolSNAP HQ interline CCD camera (Photometrics). For each slide, a mosaic of 10×10 partly overlapping images was collected with a Metamorph software (Molecular Devices) routine developed in-house. Image collections were assembled into a mosaic with the 'Stitching 2D/3D' plugin [32] (available from http://fly.mpi-cbg.de/~preibisch/software.html ) for ImageJ software (Rasband, W.S., ImageJ, US National Institutes of Health, Bethesda, Maryland, USA, http://rsb.info.nih.gov/ij/ , 1997–2009.) CDA promoter cloning and luciferase reporter assays The CDA promoter [33] was inserted into a pGL4.14 vector (Promega), upstream from the firefly luciferase gene. Cells were transfected by incubation for 72 h with 2.5 μg of the CDA promoter-containing plasmid and 0.25 μg of pGL4.74 vector (Promega, internal control, Renilla luciferase) in the presence of JetPEI reagent. Firefly luciferase and Renilla luciferase activities were assessed with the Dual-Luciferase Reporter Assay System protocol (Promega). Clonogenic survival assays Cells were plated in a drug-free medium at three different densities, in triplicate, for the counting of 30–300 clones, depending on expected survival. After 14–21 days of incubation, colonies were fixed and stained with methylene blue (5 g l −1 in 50% water and 50% methanol) and scored. Only experiments giving a linear correlation between the different dilutions were considered. Colony-forming efficiency was estimated by dividing the number of colony-forming units by the number of cells plated. Statistical analysis The significance of differences was assessed with Student's t -test or Mann–Whitney test. P <0.05 was considered statistically significant. How to cite this article: Chabosseau, P. et al . Pyrimidine pool imbalance induced by BLM helicase deficiency contributes to genetic instability in Bloom syndrome. Nat. Commun. 2:368 doi: 10.1038/ncomms1363 (2011).